Reply to: Potential contribution of PEP carboxykinase-dependent malate dismutation to the hypoxia response inC. elegans 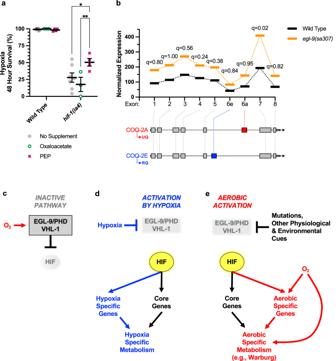Fig. 1: The hypoxia response pathway is a multifunctional context-dependent tool for regulating metabolism. aPercent of L4-stage animals surviving hypoxia (0.1% O2, 48 h at 25 °C on food, with 24 h recovery at 20 °C) after supplementation with the indicated metabolites. Error bars indicate mean ± SEM. **p= 0.0040, *p= 0.0149 ANOVA/Tukey’s multiple comparison two-sided test between each supplement and the no-supplement control.N= 7 biological replicates for untreated wild type andhif-1mutant.N= 3 biological replicates for oxaloacetate-treated wild type andhif-1.N= 4 biological replicates for PEP-treated wild type andhif-1. Although PEP partially rescuedhif-1mutants, oxaloacetate, which would hypothetically feed into the malate dismutation pathway downstream of PCK-1, did not.bDexSeq analysis of exons from the differentially splicedcoq-2gene. Isoform COQ-2A is needed to generate UQ under aerobic conditions, whereas hypoxia induces animals to switch to the COQ-2E isoform, which is needed to generate RQ for malate dismutation. No change in isoform ratio was observed inegl-9mutants versus wild type under aerobic conditions. Benjamini and Hochberg-corrected likelihood tests for individual exons are indicated byq.c–eCartoon models illustrating the multifunctional context-dependent use of the HR pathway.cUnder aerobic conditions when the pathway is not induced, EGL-9/PHD and VHL-1 use oxygen to inhibit HIF-1.dUnder hypoxic conditions, HIF-1 is disinhibited, promoting the expression of both core target genes and genes that are activated only under hypoxic conditions. The combination of these upregulated genes modulates metabolism to offset hypoxic damage.eMutations (e.g., in certain cancers) or physiological or environment cues can disinhibit HIF-1 even under aerobic conditions. HIF-1 promotes the expression of both core target genes and genes that are only activated under aerobic conditions. The combination of these upregulated genes modulates metabolism for purposes conducive for aerobic physiology (e.g., the Warburg effect). Source data are provided as a Source Data file. Hypoxia survival assays Nematodes were grown on standard NGM plates containing any indicated supplement prior to collection at the L4 stage for the assay. The supplements included 10 mM oxaloacetate (Sigma O4126) or phosphoenol pyruvic (PEP) acid trisodium salt (VWR IC15187283), which were added to NGM plates, dried at room temperature, then seeded with OP50 bacterial cultures. Garlic extract (100 μL in ethanol) was applied as a ring around the NGM agar bed to prevent nematodes from escaping the dish. L4 stage animals were added to the plates, which were then incubated at 0.1% O 2 at 25 °C for 48 h with subsequent normoxia recovery at 20 °C for 24 h. No supplement was included in recovery plates. The number of animals alive, dead, or censored (i.e., crawled out of the agar and up the edge of the dish) was counted to generate the percent survival for each trial. Thirty animals per trial were used for the assays, with the average percent of animals surviving for 48 h drawn from at least 3 independent, biological trials. Statistical analysis Simple calculations were done in MS Excel v16.70. Data for survival assays were analyzed using GraphPad Prism 9.5.1. Statistical power analysis was performed for sample size estimations using G*Power v3.1.9.6 based on our own preliminary analysis of mutants at the beginning of the study (or from previous measurements of the mutants as published), where effect size compared to wild type has been large ( d = 2.3–4.8) depending on the phenotypic assay. Researchers were blind to genotype or experimental treatment. Statistical tests were as indicated in the figure; two-sided tests were used unless otherwise indicated. Data was tested for normality using Kolmogorov-Smirnov and adjusted for multiple comparisons as indicated in the figure legends. Transcriptome analysis Previously published RNA-seq expression data from wild-type and egl-9(sa307) mutant L4 stage animals under aerobic conditions was analyzed. Reads were mapped to the C. elegans genome and transcriptome (WS273) with STAR 2.5.1a. DexSeq (v 1.28.1) was used to normalize the data and identify genes that have differential exon usage between the two genotypes (FDR < 0.05). Likelihood ratio tests for individual coq-2 exons were conducted in a pairwise fashion between genotypes with a Benjamini and Hochberg correction. RNA-seq data sets are available at NIH/NCBI GEO through accession number GSE173581. Reporting summary Further information on research design is available in the Nature Portfolio Reporting Summary linked to this article.